Plasma irregularities in the D-region ionosphere in association with sprite streamer initiation Sprites are spectacular optical emissions in the mesosphere induced by transient lightning electric fields above thunderstorms. Although the streamer nature of sprites has been generally accepted, how these filamentary plasmas are initiated remains a subject of active research. Here we present observational and modelling results showing solid evidence of pre-existing plasma irregularities in association with streamer initiation in the D-region ionosphere. The video observations show that before streamer initiation, kilometre-scale spatial structures descend rapidly with the overall diffuse emissions of the sprite halo, but slow down and stop to form the stationary glow in the vicinity of the streamer onset, from where streamers suddenly emerge. The modelling results reproduce the sub-millisecond halo dynamics and demonstrate that the descending halo structures are optical manifestations of the pre-existing plasma irregularities, which might have been produced by thunderstorm or meteor effects on the D-region ionosphere. From the Earth’s surface to its ionosphere, the planet’s atmosphere experiences an exponential decrease of its air density and an exponential increase of its electron density, leading to a transition region with unique properties in the altitude range of 60–90 km, known as the D-region of the ionosphere, between the planet’s lower atmosphere with dense air and its highly conducting ionosphere. For tropospheric thunderstorms, low electron density in this transition region enables the penetration of lightning electric fields, leading to many not yet well-understood thunderstorm effects such as electron density fluctuations and depletions [1] , [2] , as well as occasionally the formation of spectacular sprite discharges [3] . Moreover, for meteor events, the D-region is usually the lowest altitude region that meteoroids can reach owing to significant friction caused by the rapid increase of air density, resulting in plasma irregularities observed as low-altitude meteor trail echoes in radar observations [4] . Predicted in 1925 and first documented in 1989, sprite discharges originating from the D-region ionosphere have been an active research area in the past two decades [5] , [6] . Early sprite theory emphasized the importance of thunderstorm activity since it was realized soon after the discovery that intense cloud-to-ground lightning discharges associated with large charge moment changes (that is, charge times altitude from which it was removed) are necessary for their production [7] , [8] . Following that, the initiation of sprite streamers was interpreted in a modelling study as a result of the sharpening and collapse of the screening ionization wave associated with the sprite halo when the lightning charge moment change was as large as 1,300 C km (ref. 9 ). On the other hand, recent modelling studies indicate that the presence of plasma irregularities, previously thought not to be indispensable, is in fact a necessary condition for the initiation of sprite streamers [10] , [11] , in agreement with recent experimental findings showing that a large charge moment change is a necessary but not sufficient condition for sprites [12] . However, up to date, no solid evidence of D-region plasma irregularities in association with sprite streamer initiation has been presented, and if these irregularities exist their characteristics and origin(s) remain unknown. Here we show on the basis of observational and numerical modelling results that the descending halo structures recorded in the high-speed video observations, from which sprite streamers are initiated, are optical manifestation of the pre-existing plasma irregularities. An image-processing algorithm is developed to reconstruct the characteristic shape and size of those plasma irregularities, showing that sprite halos can be effectively used to probe the plasma irregularities in the D-region ionosphere. We further discuss origins of these plasma irregularities, suggesting possible relations between sprites and other thunderstorm effects or meteor events. Origin of the descending halo structures In video observations, sprite halo events exhibit a brief descending diffuse glow in the shape of a pancake with diameters up to ~80 km near ~75 km altitude, referred to as a sprite halo [13] , and develop into fine-structure filaments with diameters up to several hundred metres in the altitude range of ~40 to ~90 km, commonly referred to as sprite streamers [14] . Recent imaging of sprites at 16,000 fps indicates that before streamer initiation, spatial structures in halo emissions descend rapidly with the sprite halo, but slow down and stop to form the stationary glow in the vicinity of the streamer onset, from where streamers suddenly emerge and then accelerate exponentially [3] . The above-mentioned sub-millisecond halo dynamics is illustrated in Fig. 1 . 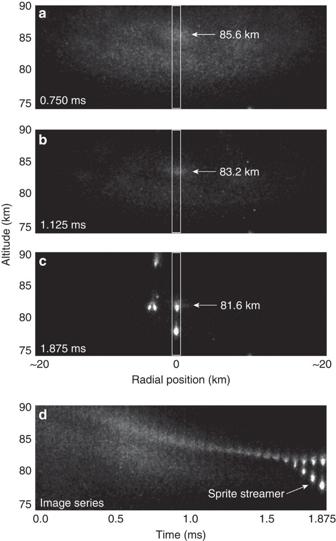Figure 1: A sprite halo event observed on 27 August 2009. The event starts at 09:15:23 085 570 UT (t=0 ms). The frame rate of the camera is 16,000 fps. Imagesaandb, respectively, show the halo emissions att=0.750 and 1.125 ms, between which the halo structure descends with an average downward speed of 6.4 × 106m s−1. Imagecshows the sprite streamer initiated from the descending spatial structure. Paneldshows a 1.875-ms image time series of the halo structure and streamer development. Figure 1: A sprite halo event observed on 27 August 2009. The event starts at 09:15:23 085 570 UT ( t =0 ms). The frame rate of the camera is 16,000 fps. Images a and b , respectively, show the halo emissions at t =0.750 and 1.125 ms, between which the halo structure descends with an average downward speed of 6.4 × 10 6 m s −1 . Image c shows the sprite streamer initiated from the descending spatial structure. Panel d shows a 1.875-ms image time series of the halo structure and streamer development. Full size image The descending halo structures appear to be of essential importance for the initiation of sprite streamers. To understand the origin of those structures, it should be first emphasized that in the transient process of halo development on a typical time scale of ~1 ms, free electrons in the lower ionosphere move only ~100 m assuming an electron drift velocity of 10 5 m s −1 , which is negligible when compared with the descending distance of halo structures on the order of ~10 km. In particular, in all halo events presented in this work, the electrons move upwards (that is, in an opposite direction to the downward movement of the halos) due to the positive polarity of the causative lightning discharges. The observed descent of a sprite halo as an entire object is due to the increase of the large-scale lightning electric field E at low altitudes and fast relaxation at high altitudes during the causative lightning discharge, leading to the lowering of the thin altitude region with large values of E / N , where N is the air density at the altitude of interest and E / N is referred to as the reduced electric field [10] . Note that large values of E / N lead to high rate of electron impact excitation of N 2 , which is the main physical process accounting for the halo optical emissions (that is, the large-scale halo is optical manifestation of the region of large reduced electric field in the lower ionosphere.) Thus, the observed descent of halo structures, proceeding at the same pace as the large-scale halo emissions, is also due to the lowering of the thin altitude region of large reduced electric field. In other words, at each moment of time, the vertical dimension of the halo structures should be defined by the vertical structuring of the reduced electric field. However, unlike its rapid spatial variation in the vertical direction, the lightning electric field varies slowly on a spatial scale of tens of kilometres in the horizontal direction, which cannot lead to the observed small-scale horizontal fluctuations in the halo optical emissions. Since the electron impact excitation rate leading to the optical emissions is determined by the reduced electric field along with the local electron density, we propose that the physical parameter that determines the horizontal dimension of the halo structures should be the fluctuations in the ambient electron density (that is, ambient plasma irregularities). To demonstrate that the downward progression of the high reduced field region and the presence of plasma irregularities can account for the observed descending halo structures, we use a two-dimensional cylindrically symmetric plasma fluid model (see Methods section) to numerically reproduce the dynamics of the descending halo structures. 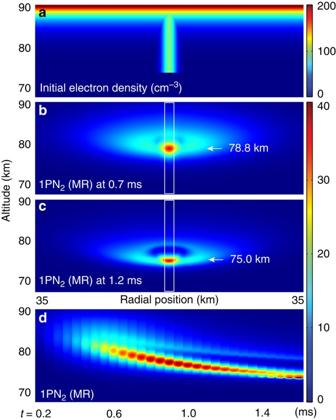Figure 2: Descending halo structure observed in a halo modelling. (a) Ambient electron density and the plasma irregularity in the simulation domain. (b,c) Halo emissions from the first positive band system of N2att=0.7 and 1.2 ms, respectively, between which the bright portion descends downward at average speed of 7.6 × 106m s−1. (d) A 1.4-ms image time series of the modelled halo structure. Figure 2a shows the ambient electron density and the plasma irregularity assumed in the simulation domain. The plasma irregularity has a Gaussian distribution in the horizontal direction with a peak value of 100 cm −3 and a characteristic size of 2 km. In the vertical direction, the plasma irregularity is homogenous and has a length of ~12 km, comparable to the descending distance of halo structures shown in Fig. 1 . Panels b and c in Fig. 2 show the sprite halo emissions from the first positive band system of N 2 at t =0.7 and 1.2 ms, respectively. It is clear that at each moment of time, only a small portion of the plasma irregularity produces emissions that are brighter than those originating from other regions of the halo. The horizontal dimension of this portion is approximately equal to the assumed horizontal size of the plasma irregularity. Examination of the spatial variation of the lightning electric field at each moment of time shows that the bright portion of the plasma irregularity is located at the altitude region with the largest reduced electric field, and the vertical dimension of the bright portion is determined by the vertical size of this altitude region. Figure 2d shows a 1.4-ms image time series of the modelled halo structure. We can see clearly that the bright potion of the plasma irregularity descends rapidly at the same pace as the remaining parts of halo emissions, but the descent slows down, and at t =1.4 ms sprite streamers start forming. The acceleration and deceleration of the descent is, respectively, due to the increase and decrease of the lightning current. The average speed of the descent (7.6 × 10 6 m s −1 ) is comparable to that of the halo structure (6.4 × 10 6 m s −1 ) shown in Fig. 1 . Figure 2: Descending halo structure observed in a halo modelling. ( a ) Ambient electron density and the plasma irregularity in the simulation domain. ( b , c ) Halo emissions from the first positive band system of N 2 at t =0.7 and 1.2 ms, respectively, between which the bright portion descends downward at average speed of 7.6 × 10 6 m s −1 . ( d ) A 1.4-ms image time series of the modelled halo structure. Full size image We note that in Fig. 2 , the streamer emerges after the halo has faded, because of a longer time scale (≥1 ms) required for streamer initiation at ~75 km altitude when compared with the duration of the halo (~1 ms for typical lightning discharges). This is consistent with the temporal relation between halo and sprite streamers revealed by the previous sprite observations [3] . It also needs to be emphasized that, although our model indicates the inception of a sprite streamer at t ≃ 1.4 ms, it cannot accurately simulate the dynamics of the sprite streamer at later moments of time owing to the low spatial resolution (~120 m) used in the large simulation domain. In the head of a streamer at ~70 km altitude, the electron density could change one order of magnitude on a spatial scale of ~2 m. This high electron density gradient requires sub-metre spatial resolution to simulate, which is beyond a practical resolution possible in a large simulation domain that uses a uniform numerical grid. Nevertheless, as shown in Fig. 2 , with a spatial resolution of ~120 m, the model is fully capable of reproducing large-scale plasma dynamics that involves only low electron density gradients, such as the experimentally observed descending halo structures. On the basis of the above analysis and comparison, it can be concluded that the halo structures are originated from pre-existing D-region plasma irregularities, and the descent of the halo structures is due to the lowering of the thin altitude region of large reduced electric field during the charge removal process of the causative lightning discharge. Reconstruction of the plasma irregularities Since at different moments of time during the lightning discharge, different portions of the plasma irregularity are effectively ‘illuminated’ by the lightning quasi-static electric field, the descending halo structures recorded by high-speed video cameras can be used to reconstruct the shape and size of the plasma irregularities in the lower ionosphere. 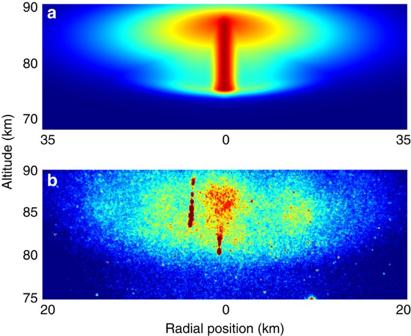Figure 3: Reconstructed plasma irregularities. (a) The plasma irregularity reconstructed using image series fromt=0 to 1.4 ms corresponding to the model event shown inFig. 2. (b) The D-region plasma irregularity reconstructed using image series of the sprite halo event shown inFig. 1. Figure 3a shows the plasma irregularity in the modelled sprite halo event reconstructed using image series from t =0 to 1.4 ms (see Fig. 2d ) and the image-processing algorithm described in the Methods. Comparison between Figs 2a and 3a indicates that the plasma irregularity in the simulation domain can be well reconstructed. Figure 3b shows the D-region plasma irregularity reconstructed using high-speed video records of the sprite halo event shown in Fig. 1 . We emphasize that the reconstructed image does not contain information about the vertical density variation, but only shows the shape and size of the plasma irregularity as manifested by optical emissions. Nevertheless, important information can be derived from it. First, sprite streamers can be easily identified because they are much brighter than the plasma irregularity and the halo. Second, the right streamer is initiated from the lower tip of the plasma irregularity. Plasma irregularity responsible for the left streamer cannot be reconstructed because if present, it should be located above the available field of view of the camera. Third, the size of the plasma irregularity can be estimated using two different approaches. On the basis of the altitude range of the entire image, which is calculated assuming the sprite streamer was directly above the causative lightning discharge, the vertical and horizontal size of the plasma irregularity are, respectively, ~5 and ~1 km. Alternatively, based on a 100-m typical diameter of sprite streamers documented in the existing literature [15] , the vertical and horizontal size of the plasma irregularity are, respectively, ~2.5 and ~0.5 km. These two estimates are roughly consistent with each other. Note that it is possible that the plasma irregularity has a significantly longer vertical dimension than that revealed in Fig. 3b , because the lightning electric field cannot penetrate into higher altitudes so that even if a significant portion exists at high altitudes, it cannot be ‘illuminated’. Figure 3: Reconstructed plasma irregularities. ( a ) The plasma irregularity reconstructed using image series from t =0 to 1.4 ms corresponding to the model event shown in Fig. 2 . ( b ) The D-region plasma irregularity reconstructed using image series of the sprite halo event shown in Fig. 1 . Full size image To further demonstrate the characteristics of plasma irregularities in association with sprite streamer initiation, we analyse another sprite halo event observed on 20 July 2012 in which multiple plasma irregularities can be identified in the halo. For this event, the halo emissions first appear at 06:27:17:157 860 UT ( t =0 ms). 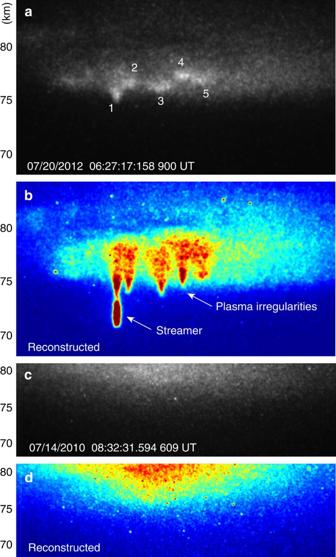Figure 4: Halo events with and without plasma irregularities. (a,b) A frame of the sprite halo event observed on 20 July 2012 and the reconstructed image showing five plasma irregularities. (c,d) A frame of the halo event observed on 14 July 2010 and the reconstructed image that shows only large-scale halo emissions. Figure 4a shows the halo emissions at t =1.04 ms. Five bright halo structures are identifiable at this moment of time, and in the video record they all experience descending motion similar to that shown in Fig. 1d . At t =1.28 ms, a sprite streamer was already initiated from the leftmost halo structure. For all the other four halo structures, t =1.28 ms is the moment just before the initiation of sprite streamers. Figure 4b shows the five plasma irregularities reconstructed using all video frames from t =0 to 1.28 ms. These plasma irregularities are, respectively, responsible for the five descending halo structures (see Fig. 4a ) and the following five sprite elements (not all shown in Fig. 4b ). As an additional evidence, Fig. 4c shows a halo event with no following sprite streamers. This halo event was observed on 14 July 2010 starting at 08:32:31.594 409 UT, and it has a typical pancake shape, which is defined by the spatial variation of the large-scale lightning electric field. In the reconstructed image shown in Fig. 4d , no plasma irregularities and sprite streamers can be identified, which is an indirect evidence suggesting the importance of plasma irregularities for the initiation of sprite streamers. Figure 4: Halo events with and without plasma irregularities. ( a , b ) A frame of the sprite halo event observed on 20 July 2012 and the reconstructed image showing five plasma irregularities. ( c , d ) A frame of the halo event observed on 14 July 2010 and the reconstructed image that shows only large-scale halo emissions. Full size image A recently proposed theory suggests that the presence of strong plasma irregularities in the D-region ionosphere is a necessary condition for the initiation of sprite streamers [10] , [16] , and modelling results show that vertically elongated plasma columns are more favourable for streamer initiation when compared with spherical irregularities [17] , [18] . The above reconstructed images demonstrate for the first time solid evidence of kilometre-scale plasma irregularities in association with sprite streamer initiation in the D-region ionosphere. However, it is important to emphasize that not all the plasma irregularities in association with sprite streamer initiation can be observed as descending halo structures in video records of sprite events. Two reasons can lead to the absence of descending halo structures in sprite observations. First, the descending halo structures emphasized in the present work are due to a significant vertical dimension of the plasma irregularities leading to the effective illumination of a small portion of the plasma irregularities at each moment of time by the lightning electric field. In the case when the plasma irregularities are approximately spherical and have a compact size of tens to hundreds of metres, which are capable of initiating sprite streamers according to the previous modelling studies [16] , [19] , the plasma irregularities could only be recorded as a local enhancement of the halo luminosity around the origin of sprite streamers. Second, the brightness of halos depends on the impulsiveness of the causative lightning discharges [19] . In some sprite events, the halo and halo structures can remain sub-visual if the charge transferring lightning current is not impulsive enough. We note that a relatively bright but not saturated large-scale halo is ideal for the reconstruction of the plasma irregularities. It has also been verified that in some cases when only the descending halo structures are visible, the reconstruction is also possible since halo structures are brighter than the other parts of the halo, which remain sub-visual. According to previous modelling studies [11] , [17] , [19] , the electron density in plasma irregularities needs to be ~2–5 orders of magnitude higher than the ambient electron density to initiate sprite streamers, depending on the onset altitude of the sprite streamers (at lower altitudes, the difference needs to be larger). It is reasonable to believe that such strong perturbations cannot persist in a quiet lower ionosphere, and it is important to emphasize that the origin(s) of those plasma irregularities cannot be determined using the results presented in this work. The several possible origins are discussed below. Tropospheric thunderstorms are well known to be able to disturb the lower ionosphere by convective atmospheric gravity waves and by lightning electric fields, leading to conductivity enhancement, electron density depletions and D-layer reflection height splitting [1] , [2] , [7] , [20] . However, most of those are large spatial scale processes. One possible thunderstorm effect that could produce the kilometre-scale plasma irregularities with a density enhancement of at least ~2 orders of magnitude is sprites themselves. Previous modelling results suggest that the electron density enhancement in sprite bodies can typically last for ~100 s at ~75 km altitude [21] . The remnant of a previous sprite body could indeed facilitate the initiation of sprites at tens of milliseconds later according to video observations [22] , [23] . To examine the possibility of previous sprites producing the plasma irregularities observed in Figs 1 and 4a , we have analysed the images of sprites captured before those events on the same nights. We find that no previous sprites occurred at the same location as the one shown in Fig. 1 . For the event shown in Fig. 4a , a sprite event occurred ~10 min before, and the bright sprite columns captured by the same camera largely overlap with the sprites shown in Fig. 4a . Unfortunately, images captured using another camera missed most parts of the two events so that the exact coincidence of the sprite locations cannot be verified using a triangulation technique. The ~10 min time separation is much longer than the ~100 s relaxation time of the electron density enhancement at ~75 km altitude estimated in modelling of sprite chemistry [21] . On the other hand, recent coordinated radio and optical observations show that long recovery early very low frequency (VLF) events, caused by long-lasting (a few hundred seconds to tens of minutes) D-region ionospheric conductivity modifications, occurred often coincidently with bright sprites [24] . It has been suggested that the long-lasting conductivity modifications may have been produced by those concurrent sprites [24] . Although how the electron density enhancement in sprites could last so long is not clear, the plasma irregularities shown in Fig. 4a might be related to the previous sprite event that occurred ~10 min before. Considering the requirement of several orders of magnitude plasma density enhancement for streamer initiation, those plasma irregularities might have been produced by meteor events. Meteors had been suggested to be a possible factor for the initiation of sprite streamers in early sprite research, but soon the idea was discarded because using a visually observed meteor flux density of 8 × 10 −7 km −2 s −1 it was estimated that for a sprite with a horizontal cross-sectional area of ~175 km 2 one would expect only ~10 −4 sporadic meteors to intersect a sprite volume in a 1-s interval before the optical observation of the sprite [25] . However, radar observations show that visual and sub-visual meteors are continuously entering the Earth’s upper atmosphere with a much larger flux density estimated to be ~10 −4 km −2 s −1 globally [26] . Moreover, the entire volume of a large-scale halo, which covers a horizontal cross-sectional area of assuming a radius R halo of 40 km, should be used in the estimate because sprites could have lateral offsets as large as ~40–50 km with respect to the causative lightning discharge [27] . With these different values and assuming that 10% of the meteoroids could reach the sprite altitudes, it is estimated that on average 0.05 meteors could intersect a large-scale halo volume in a 1-s interval before sprite initiation. We note that the above estimate is rough as no observations are yet available quantifying the meteor flux density in a specific region above an active sprite-producing thunderstorm. Nevertheless, this estimate suggests a higher probability (that is, 5% using the methodology described above) of a positive correlation between sprite and meteor events than that shown in previous literature. In summary, a comparison of experimental and numerical results presented in this study demonstrates that the descending halo structures in sprite halo events recorded by high-speed video cameras are the optical manifestation of pre-existing plasma irregularities in the D-region ionosphere. It is the first time that robust evidence of plasma irregularities in association with sprite streamer initiation has been presented and the characteristic size of these plasma irregularities quantified. Thunderstorm effects and meteor events are suggested to be two possible origins of these plasma irregularities. We note that future observations focusing on halo structures and modelling studies are necessary to understand the origin(s) of these D-region plasma irregularities in association with sprite initiation. Plasma fluid model In our plasma fluid model [19] , the chemical reactions accounted for include the electron impact ionization of N 2 and O 2 , the electron dissociative attachment to O 2 and the electron detachment process O − +N 2 →e+N 2 O. Note that, although included, the effect of detachment in our simulations is negligible over a ~2 ms time scale. Photoionization processes are included using the three-group SP 3 model [28] . The motion of charged species is simulated by solving the drift-diffusion equations for electrons and ions coupled with Poisson’s equation [19] . The transport equations for charged species are solved using a flux-corrected transport technique that combines an eighth-order scheme for the high-order fluxes and a donor cell scheme for the low-order fluxes. The simulation domain extends from ground up to 95 km, has a radius of 95 km and is discretized using a grid with a spatial resolution of ~120 m. It is assumed that perfectly conducting boundary conditions are satisfied on all boundaries of the simulation domain. Ambient electron density profile The ambient electron density profile can be expressed as [29] : where h ′ (km) and β (km −1 ) are given parameters describing reference altitude and sharpness, respectively. We assume that h ′=85 km and β =0.5 km −1 , which represent a typical nighttime electron density profile. The positive ion density n ion is assumed to be equal to the electron density at high altitudes where electron density has values larger than 10 8 m −3 , and at lower altitudes the positive ion density is equal to 10 8 m −3 . Initial ambient negative ion density is then calculated based on charge neutrality. Lightning current waveform The waveform for lightning current moment is modelled using the following formulation [30] : where the lightning charge moment change Qh Q is chosen to be 800 C km and t 0 =25 μs that corresponds to a lightning discharge with a duration of ~1 ms. The image-processing algorithm To reconstruct the shape and size of the plasma irregularities, different image-processing algorithms could be developed. Here we provide an illustration of a simple and effective algorithm developed as part of the present work. All frames from the beginning of the halo to streamer initiation are used in the reconstruction process. First, each frame is converted to an 8 bit grey scale image. Second, the intensity in each image is linearly normalized to equalize the peak intensity in different images. The purpose of this normalization is to make the brightness of the halo structures in different images that correspond to different portions of the plasma irregularities comparable. The rationale of the normalization is explained as follows. The brightness of the halo structures in the original image time series could be significantly different from each other. This difference is mainly due to the temporal variation of the reduced electric field (see for example, Fig. 1 in ref. 16 ), and may partially stem from vertical density variation in the plasma irregularities. In other words, difference in the brightness of the halo structures in different images does not necessarily indicate that the density in the body of a plasma irregularity varies significantly in the vertical dimension. As shown in Fig. 2d , even if the plasma irregularity is assumed to be vertically homogenous, temporal variation of the lightning electric field could still lead to significant difference in the brightness of the halo structure. Since our aim is to reconstruct the shape and size, rather than the density variation of the plasma irregularities, we remove the effect of lightning electric field variation by equalizing the peak intensity in the sprite images. This step is important as otherwise some parts of the plasma irregularities cannot always be reconstructed owing to weak brightness when compared with other parts. In the final step, we compare the normalized images pixel by pixel retaining only the maximum intensity in each pixel and using these values to form the reconstructed image. Assuming that 10 normalized images are used in the reconstruction, and each has a total number of pixels M × N. For each pixel denoted by ( m , n ), there are 10 different intensity values I ( m , n ) from those 10 normalized images, among which the maximum one I max ( m , n ) is chosen to be the intensity in the pixel ( m , n ) of the reconstructed image. Using this algorithm, the halo structures captured in an image time series can be merged in a single image to reveal the shape and size of the plasma irregularities. How to cite this article: Qin, J. et al. Plasma irregularities in the D-region ionosphere in association with sprite streamer initiation. Nat. Commun. 5:3740 doi: 10.1038/ncomms4740 (2014).